A Gondwanan imprint on global diversity and domestication of wine and cider yeastSaccharomyces uvarum In addition to Saccharomyces cerevisiae , the cryotolerant yeast species S. uvarum is also used for wine and cider fermentation but nothing is known about its natural history. Here we use a population genomics approach to investigate its global phylogeography and domestication fingerprints using a collection of isolates obtained from fermented beverages and from natural environments on five continents. South American isolates contain more genetic diversity than that found in the Northern Hemisphere. Moreover, coalescence analyses suggest that a Patagonian sub-population gave rise to the Holarctic population through a recent bottleneck. Holarctic strains display multiple introgressions from other Saccharomyces species, those from S. eubayanus being prevalent in European strains associated with human-driven fermentations. These introgressions are absent in the large majority of wild strains and gene ontology analyses indicate that several gene categories relevant for wine fermentation are overrepresented. Such findings constitute a first indication of domestication in S. uvarum. The budding yeast Saccharomyces cerevisiae has been used for millennia by humans for the fermentation of foods and beverages [1] , [2] . This association is the foundation of its use as a model organism in various areas of biological research, including molecular genetics, biomedicine, biotechnology and, more recently, evolutionary genomics [3] . For decades, the natural biology of S. cerevisiae remained elusive, but a better understanding of its natural habitats [4] and distribution [5] , combined with the widespread use of whole-genome data [6] , [7] , [8] , [9] , are providing a new ecological framework for the understanding of the diverse cellular, molecular and evolutionary mechanisms that shaped the world’s most biotechnologically important microbe. As a consequence, renewed attention is being paid to the importance of field work for capturing unknown genetic diversity and for gathering quantitative ecological data [5] , [10] . Natural Saccharomyces species distinct from S. cerevisiae are not frequently associated with human-driven fermentations, but several are often found as contributors to interspecies hybrids used in beer and wine production. In fact, the most economically important industrial yeast after S. cerevisiae is the polyploid hybrid S. pastorianus , which is used in brewing lager beer. S. pastorianus is the result of domestication associated with brewing at low temperatures and combines the genome of a S. cerevisiae ale yeast with that of the recently described cryotolerant yeast S. eubayanus [11] , [12] . Other hybrids harbouring genomic contributions from S. cerevisiae and a distinct cryotolerant species, S. kudriavzevii , are commonly found among strains used to produce Belgian-style beers and wines fermented at low temperatures [13] , [14] , [15] . It now seems clear that, in low-temperature fermentations, S. cerevisiae generally tends to be replaced by hybrids that combine the genomes of S. cerevisiae with those of S. eubayanus, S. kudriavzevii and S. uvarum , a third cryotolerant species. S. uvarum occupies a basal position in the Saccharomyces phylogeny, sister to S. eubayanus , making the two species the most distantly related to S. cerevisiae within the genus. Unlike S. eubayanus, S. uvarum does not contribute to the genome of lager-brewing strains but rather stands out as the only natural, non-hybrid species other than S. cerevisiae that is relevant for industrial fermentations. S. uvarum has a fermentation profile in grape must that is different from that of S. cerevisiae , producing less acetic acid and ethanol but more glycerol and succinic acid, while synthesizing malic acid without posterior degradation [16] , [17] , [18] . Moreover, S. uvarum produces volatile fermentative compounds such as phenylethanol and its acetate [19] or volatile thiols [20] . These phenotypic differences between S. uvarum and S. cerevisiae are associated with pronounced proteomic differences [21] . The wines typically fermented by S. uvarum are Tokaj (Hungary, Slovakia), Amarone (Italy), and Txakoli (Spain); and in France, Sauternes and the whites of northern French vineyards in Burgundy, Champagne, Val de Loire and Alsace [22] , [23] , [24] , [25] , [26] , [27] . S. uvarum is also frequently responsible for cider fermentation, which is usually conducted at low temperatures [28] , [29] . Little information is available on the distribution of S. uvarum , and virtually nothing is known concerning possible domestication events. Apart from the appreciable number of strains that have been isolated in Europe from fermentations, only a few strains from natural environments have been obtained in Europe and North America, mostly in association with oak trees [4] . Interestingly, a radically different situation was encountered in South America. After extensive fieldwork on Nothofagus (southern beech), a tree genus that, along with Quercus (oaks), belongs to the order Fagales, we discovered a conspicuous population of S. uvarum in sympatry with S. eubayanus in Patagonia [12] . Such findings encouraged us to obtain a more representative strain data set of S. uvarum , especially in Australasia, the only other region of the globe where Nothofagus are native. Here we describe the use of a population genomics approach to perform a comprehensive phylogeographic survey of S. uvarum with special focus on the detection, for the first time, of fingerprints of domestication in this species. Occurrence of S. uvarum in the Southern Hemisphere We previously reported the sympatric occurrence of a wild population of S. uvarum and its novel sibling species S. eubayanus in Northwestern Patagonia, in association with Nothofagus and the sugar-rich fruiting structures (stromata) of its biotrophic fungal parasite, Cyttaria hariotii [12] . In that study, 47 isolates of S. uvarum were recovered from 133 samples obtained from three species of Nothofagus , with N. dombeyi standing out as the species with the highest frequency of isolation with a global success rate of 35%. A much lower frequency of isolation had been previously obtained for this species in Europe when the Quercus habitat was explored [4] . This difference prompted us to study the ecological association of S. uvarum with the Nothofagus–Cyttaria system, not only in Patagonia but also in Australasia. Therefore, we carried out an expanded survey that included a southward extension of the Patagonian region previously covered, as well as sampling in Australia and New Zealand. In the South American survey, 218 samples that included N. dombeyi and five additional species of Nothofagus were collected in the Spring and Summer months of 2008, 2009 and 2010, yielding 59 S. uvarum isolates. In Australasia, 113 samples were collected in the Spring of 2009, yielding eight isolates. To provide insight into the global genetic diversity and phylogeography of S. uvarum , a set of strains representing the entire scope of geographic origins and habitats ( Fig. 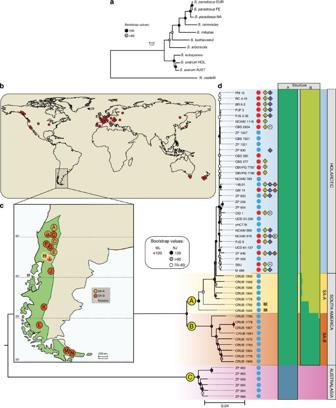Figure 1: Geographic distribution, phylogeny and population structure ofS. uvarum. (a) Maximum likelihood (ML) phylogeny of the genusSaccharomycesbased on a concatenated alignment of 14 gene sequences and rooted withN. castellii. Representatives of populations ofS. paradoxus(EUR, European; FE, Far Eastern; and NA, North American) and of the Australasian (AUST) and Holarctic (HOL) populations ofS. uvarumare included. Support values correspond to 100 bootstrap replicates and branch lengths correspond to the mean number of nucleotide substitutions per site. (b) World map depicting the geographic origin of HOL and AUSTS. uvarumstrains. (c) Map of South America depicting the collecting sites. Locations are indicated by capital letters surrounded by light- or dark-orange coloured circles corresponding to populations SA-A and SA-B, respectively. The co-occurrence of strains of the two populations is depicted by light- and dark-orange semi-circles, and the occurrence of mosaic strains is depicted by white contour lines. The distribution ofNothofagusis shown in green. (d) Whole-genome Neighbor-Joining (NJ) phylogeny of 54 strains based on 129,096 SNPs and excluding introgressed regions fromS. eubayanus, inferred withp-distance and rooted withS. eubayanus. The three main clades are marked by letters A, B and C. Support values from 1,000 bootstrap NJ and ML (RAxML rapid bootstrap) trees are included. Incongruent topologies between NJ and ML are denoted by grey lines. Branch lengths correspond to the mean number of base differences per site. Strains isolated from natural environments are marked by blue circles, whereas strains isolated from anthropic environments are marked by red circles. Strains having introgressions are marked with an ‘I’ in a yellow (introgressions fromS. eubayanus), blue (introgressions fromS. kudriavzevii) or orange (introgressions fromS. cerevisiae) diamond. For the hybrid strains (marked with an ‘H’ in a white circle) orS. bayanus(‘B’ in a white circle), only introgressions in theS. uvarumsub-genome are depicted. South American mosaic strains are marked with an ‘M’ in an orange square. Clusters inferred with STRUCTURE considering all sequences (A) and all but the Australasian sequences (B) are depicted. 1b,c and Supplementary Table 1 ) was selected for whole-genome sequencing using the Illumina technology. In addition to a representative collection of isolates from the Nothofagus niche, our strain data set also included wild isolates collected in North America, Eurasia and Far East Asia, which was obtained mostly from the bark of oak trees and associated soil. In addition, European strains isolated from artificial environments, mostly wine and cider, were included. Finally, three confirmed hybrid strains of S. uvarum × S. cerevisiae (two of them, triple hybrids with contributions also from S. kudriavzevii ) were also included ( Supplementary Table 1 ). The phylogenetic relationships of 54 strains, based on 129,096 high-quality polymorphic sites, are depicted in Fig. 1d ( Supplementary Fig. 1 depicts a topologically similar phylogeny obtained on an expanded set of 61 strains using 3,113 high-quality single-nucleotide polymorphisms (SNPs) from chromosomes 5, 8 and 12). This broad phylogenetic analysis resolved the various representatives of S. uvarum into three main clades. Clade A contained all Holarctic strains and a few from South America; clade B encompassed only strains from South America; and clade C corresponded to the Australasian population and was clearly separated from the other two clades. In fact, this lineage was 4.4% divergent (divergence per site, k , with Jukes–Cantor correction) from the other two main lineages, which is similar to the divergence of the North American population of S. paradoxus from both the European and Far Eastern populations [30] . In spite of their divergence, the Australasian strains are clearly more closely related to S. uvarum than to any other Saccharomyces species, as depicted in Fig. 1a . The phenotypic profiling of the Australasian isolates showed also some unique features, including delayed or absent growth on maltose and melibiose, maximum growth temperatures 3–4 °C lower than those observed for other S. uvarum strains (31–32 versus 35 °C for the non-Australasian strains), and lower growth rates on melibiose at some temperatures ( Supplementary Tables 2 and 3 ). Figure 1: Geographic distribution, phylogeny and population structure of S. uvarum . ( a ) Maximum likelihood (ML) phylogeny of the genus Saccharomyces based on a concatenated alignment of 14 gene sequences and rooted with N. castellii . Representatives of populations of S. paradoxus (EUR, European; FE, Far Eastern; and NA, North American) and of the Australasian (AUST) and Holarctic (HOL) populations of S. uvarum are included. Support values correspond to 100 bootstrap replicates and branch lengths correspond to the mean number of nucleotide substitutions per site. ( b ) World map depicting the geographic origin of HOL and AUST S. uvarum strains. ( c ) Map of South America depicting the collecting sites. Locations are indicated by capital letters surrounded by light- or dark-orange coloured circles corresponding to populations SA-A and SA-B, respectively. The co-occurrence of strains of the two populations is depicted by light- and dark-orange semi-circles, and the occurrence of mosaic strains is depicted by white contour lines. The distribution of Nothofagus is shown in green. ( d ) Whole-genome Neighbor-Joining (NJ) phylogeny of 54 strains based on 129,096 SNPs and excluding introgressed regions from S. eubayanus , inferred with p -distance and rooted with S. eubayanus . The three main clades are marked by letters A, B and C. Support values from 1,000 bootstrap NJ and ML (RAxML rapid bootstrap) trees are included. Incongruent topologies between NJ and ML are denoted by grey lines. Branch lengths correspond to the mean number of base differences per site. Strains isolated from natural environments are marked by blue circles, whereas strains isolated from anthropic environments are marked by red circles. Strains having introgressions are marked with an ‘I’ in a yellow (introgressions from S. eubayanus ), blue (introgressions from S. kudriavzevii ) or orange (introgressions from S. cerevisiae ) diamond. For the hybrid strains (marked with an ‘H’ in a white circle) or S. bayanus (‘B’ in a white circle), only introgressions in the S. uvarum sub-genome are depicted. South American mosaic strains are marked with an ‘M’ in an orange square. Clusters inferred with STRUCTURE considering all sequences (A) and all but the Australasian sequences (B) are depicted. Full size image The observation that the Australasian strains were both genetically and phenotypically divergent from the remaining lineages, combined with their geographic isolation, led us to hypothesize that the observed divergence could be the consequence of allopatric partitioning. To help ascertain this, we performed crosses between Australasian strains and representatives of the other two main lineages represented in Fig. 1d and determined the viability of the resulting progeny. Interestingly, the four crosses involving an Australasian strain mated with a South American or European strain yielded intermediate levels of spore viability of 27–36% ( Supplementary Table 4 ), whereas the progeny of the cross of two Australasian strains, one from Tasmania and the other from New Zealand, had 95.7% spore viability. Another observation worth noting was the relatively high spore viability (18.8%) produced by a cross between an Australasian S. uvarum representative and a South American strain of S. eubayanus ( Supplementary Table 4 ). 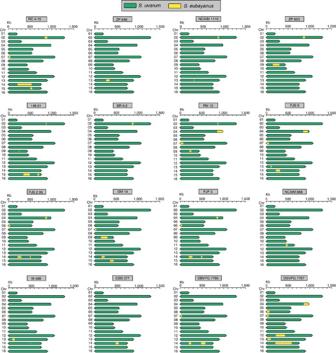Figure 4: Chromosome maps ofS. uvarumstrains showing the location and extent of introgressions fromS. eubayanus. The maps are shown for the 16 strains that haveS. eubayanusintrogressions (hybrid strains excluded). This value contrasts with the reported 7% of spore viability from crosses of sympatric (South American) representatives of S. uvarum and S. eubayanus [12] , which could be a sign of the reinforcement of reproductive isolation that deserves further study. Population structure and phylogeography in South America The S. uvarum phylogeny ( Fig. 1d ) revealed that, by far, most of the diversity contained in this species is found in the Southern Hemisphere. In fact, the nucleotide diversity based on pairwise differences ( π × 100) contained in the group of South American isolates was 0.689, approximately half of the nucleotide diversity observed globally for the species (1.248) and much higher than that of the Australasian isolates (0.162) and of the Holarctic group (0.141; Supplementary Table 5 ). Therefore, in addition to the extremely divergent Australasian lineage, the isolates from the Southern Hemisphere encompass more genetic diversity than those from the Northern Hemisphere. This high diversity observed for the Patagonian strains can be partly attributed to the presence of two major well-separated lineages, such as clades A and B. The South American strains of clade A (SA-A) are phylogenetically related to the Northern Hemisphere group and were placed at the basal positions of this branch, whereas the Holarctic isolates occupied more nested positions ( Fig. 1d ). Clade B was restricted to South American strains only, and is hereafter designated SA-B. The two South American lineages (SA-A and SA-B) had a genetic distance of 1.0% ( Supplementary Table 6 ) and genetic diversities of 0.415 (SA-A) and 0.333 (SA-B) ( Supplementary Table 5 ). Population structure inference carried out in STRUCTURE ( Fig. 1d ) clearly indicated the presence of two distinct genetic clusters in our worldwide sampling, as determined by the high value of the ad hoc statistic, Δ K , which measures the rate of change between log probabilities for successive K values (Δ K 2 =3682.6). One of these clusters was assigned to the Australasian lineage and the other consisted of all remaining isolates (South America and Holarctic region). Because STRUCTURE inference is strongly influenced by the sampled genotypes that are used to run the software and because of the marked divergence of the Australasian population, we excluded this lineage from the data set and repeated the analysis. Interestingly, this restricted S. uvarum data set was resolved into two new genetic clusters that reflected our phylogenetic inference, one cluster was cosmopolitan and present in both South America and the Northern Hemisphere, whereas the other cluster was endemic to South America (SA-B; Fig. 1d ). Increasing values of K suggested only minor possible ancestry contributions to those two clusters and did not uncover any new clean clusters ( Supplementary Fig. 2 ). In addition to the strains clearly belonging to either one of these two populations, there were also two strains in the phylogenetic tree (CRUB 1782 and CRUB 1595) that occupied positions that could be explained by a mosaic structure of their genomes, with contributions from different lineages. In fact, these strains showed mixed ancestries in STRUCTURE ( Fig. 1d ), which is consistent with admixture between the two populations. A sliding window analysis comparing the genome of CRUB 1782 with those of strains representing each of the two clean lineages confirmed that it was nearly identical to one or the other of the two South American populations across its genome ( Supplementary Fig. 3 ). These analyses suggested that both strains were ~65% SA-A and 35% SA-B, although the exact regions contributed by each parental population were frequently non-overlapping. The existence of strains with mixed ancestries is in line with the high (97%) spore viability found in crosses between strains representing the two populations ( Supplementary Table 4 ). Limited genetic diversity of the Holarctic population When compared with the genetic diversity observed for strains from the Southern Hemisphere, strains from a wide range of environments in the Northern Hemisphere show remarkably low diversity across their genomes. This seems to be consistent with the Southern Hemisphere and the Nothofagus–Cyttaria system being native geographical ranges and habitats of S. uvarum , respectively. It also suggests the hypothesis of a recent migration of the Patagonian S. uvarum population SA-A into the Northern Hemisphere and the consequent habitat shift to oaks and other non- Nothofagus trees imposed by the absence of Nothofagus north of the equator. Indeed, several lines of evidence support the view that the Northern Hemisphere population might be recently derived from the South American SA-A population. First, the nucleotide diversity is much higher in the SA-A population (0.00415) than in the Holarctic population (0.00141), as shown in Supplementary Table 5 . In addition, the Holarctic group has the highest value of Tajima’s D statistic, although it is not significant. The relative excess of intermediate frequency alleles is compatible with a recent population contraction where there has not been sufficient time for many new mutations to accumulate ( Supplementary Table 5 ). Moreover, the analysis of shared polymorphisms involving the South American and Holarctic populations supports the hypothesis that the Northern Hemisphere population is derived from the Patagonian SA-A population. The proportion of shared polymorphisms between the SA-A and Holarctic populations is much higher than that of the comparison involving SA-B and Holarctic populations ( Fig. 2 ). In addition, an almost negligible proportion of fixed differences were found between the SA-A and Holarctic populations, contrary to what was observed between SA-A and SA-B and, most notably, between the Holarctic population and SA-B. If the Northern Hemisphere population has derived from the Patagonian SA-A population, the time to coalescence of all Holarctic lineages in a single common ancestor is expected to be more recent than that of the coalescence of lineages of SA-A. In fact, an analysis of relative coalescence times suggested a more recent common ancestor for the Northern Hemisphere population than for either of the South American populations. Specifically, the Holarctic clade is only ~71% as old as the SA-A clade ( Fig. 2 ), which fits in a model of colonization of the Northern Hemisphere from South America. Therefore, taken together, our analyses support the view suggested by the phylogeny in Fig. 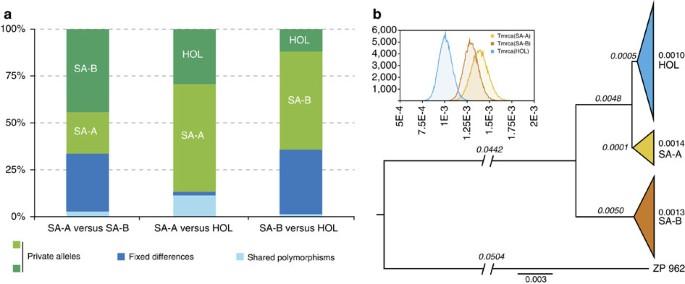1d that the Northern Patagonian population SA-A gave rise to the Holarctic population. Figure 2: Proportion of shared and privately segregating polymorphisms and coalescence analysis in the South American and Holarctic (HOL) populations. (a) Proportion of private alleles, fixed differences and shared polymorphisms among SNPs found in all possible pairwise comparisons involving the HOL and the two South American populations, SA-A and SA-B (South American mosaic strains were excluded from the analysis). (b) Genome-wide estimation of relative time to coalescence for the HOL and the two South American populations. The tree was built from an alignment of 51,159 high-quality sites (Phred quality score >Q40) partitioned over the 16 chromosomes. Each partition represents regions without evidence for intra-locus recombination. The scale bar depicts estimated substitutions per site. Node ages are printed in bold near the nodes of the population whose coalescence they estimate. Branch lengths are printed in italics above the branches. One representative strain of the divergent Australasian population was used to root the tree. The insert shows the marginal posterior densities of the time to the most recent common ancestor (tmrca) in each population. Figure 2: Proportion of shared and privately segregating polymorphisms and coalescence analysis in the South American and Holarctic (HOL) populations. ( a ) Proportion of private alleles, fixed differences and shared polymorphisms among SNPs found in all possible pairwise comparisons involving the HOL and the two South American populations, SA-A and SA-B (South American mosaic strains were excluded from the analysis). ( b ) Genome-wide estimation of relative time to coalescence for the HOL and the two South American populations. The tree was built from an alignment of 51,159 high-quality sites (Phred quality score >Q40) partitioned over the 16 chromosomes. Each partition represents regions without evidence for intra-locus recombination. The scale bar depicts estimated substitutions per site. Node ages are printed in bold near the nodes of the population whose coalescence they estimate. Branch lengths are printed in italics above the branches. One representative strain of the divergent Australasian population was used to root the tree. The insert shows the marginal posterior densities of the time to the most recent common ancestor (tmrca) in each population. Full size image Introgressions from other Saccharomyces species Since several introgression events were previously reported between S. paradoxus and S. cerevisiae [30] , [31] , [32] , [33] , [34] , we screened the genome sequences for introgressions from other Saccharomyces species. Although signs of foreign genomic DNA were not found in strains isolated in the Southern Hemisphere, 20 out of 34 Holarctic strains displayed multiple introgressions that could be clearly ascribed to various Saccharomyces species, including from S. kudriavzevii (14 strains), S. cerevisiae (3 strains) and most notably from S. eubayanus (20 strains; Supplementary Data 1 and 2 ). These introgressions were widespread across the S. uvarum genomes, but their number and size were found to differ between strains. The precise locations and distributions of the introgressions are summarized in Figs 3 and 4 . Interestingly, all but one of the 18 strains isolated from anthropic niches were found to have introgressions, either solely from S. eubayanus or from up to two additional Saccharomyces species ( Fig. 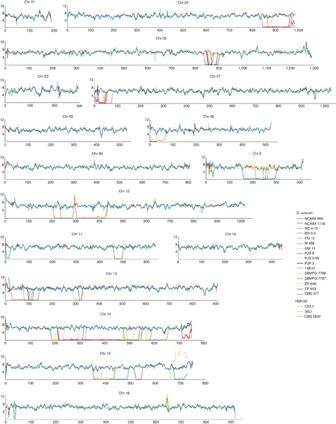1d and Supplementary Data 1 ). Figure 3: Sliding window analysis ofS. eubayanusintrogressions inS. uvarumgenomes. Each plot represents the % divergencek(with Jukes–Cantor correction) relative toS. eubayanusreference strain CRUB 1568 (x-axis values are in Kb). Introgressed strains are color-coded according to the key. Figure 3: Sliding window analysis of S. eubayanus introgressions in S. uvarum genomes. Each plot represents the % divergence k (with Jukes–Cantor correction) relative to S. eubayanus reference strain CRUB 1568 (x-axis values are in Kb). Introgressed strains are color-coded according to the key. Full size image Figure 4: Chromosome maps of S. uvarum strains showing the location and extent of introgressions from S. eubayanus . The maps are shown for the 16 strains that have S. eubayanus introgressions (hybrid strains excluded). Full size image The most striking and recurrent introgressions are from S. kudriavzevii and S. eubayanus. The S. kudriavzevii introgressions are all partially overlapping and relatively short (encompassing up to seven genes). Sequence comparison readily shows that these fragments of S. kudriavzevii DNA were acquired from the European population of the species, in line with the European origin of all but one of the strains harbouring the S. kudriavzevii introgressions. Curiously, the sole non-European strain carrying a S. kudriavzevii introgression was isolated in Japan, where a genetically distinct S. kudriavzevii population has been identified [33] . However, this strain is likely to be phylogenetically related with the European strains since its S. kudriavzevii introgression is very similar to those present in European strains, both in gene content and sequence ( Supplementary Data 1 ). Introgressions from S. eubayanus are the most prevalent and extensive. The introgressions are, on average, 99.5% identical to the genome of the South American strain of S. eubayanus CRUB 1568 (FM1318), but they are 99.9% identical to the S. eubayanus portion of the genome of S. pastorianus strain Weihenstephan 34/70. This divergence between the S. eubayanus type strain and the S. eubayanus moiety found in S. pastorianus has already been reported [12] . Since all the S. uvarum strains with S. eubayanus introgressions are European, it seems reasonable to assume that the introgressions occurred in Europe. Therefore, these results suggest that the S. eubayanus introgressions in S. uvarum either originate from S. pastorianus or are derived from a yet-unidentified Eurasian lineage of S. eubayanus that was also the contributor to the genomes of the hybrid species S. pastorianus and S. bayanus . The number of S. eubayanus introgressions per strain varied between seven (strain DBVPG 7787) and one (strains CBS 377, BR 6-2, NCAIM 868, ZP 646 and CID 1). The genes involved in the introgressions are listed in Supplementary Data 2 , excluding those present in strain NCAIM 676, which possesses a much more extensive contribution from S. eubayanus . This strain has a genomic composition similar to that of S. bayanus strains CBS 380 and NBRC 1948 ( Supplementary Table 7 ). NCAIM 676 has slightly more genetic material from S. uvarum than from S. eubayanus , but the extensive genomic contributions from S. eubayanus and limited contributions from S. cerevisiae suggest that it should be regarded as a representative of the artificial species S. bayanus sensu Libkind et al [12] . The S. uvarum hybrids CBS 2834, CID 1 and S6U contain substantial contributions across their genomes from S. cerevisiae and/or S. kudriavzevii ( Supplementary Table 7 ). We searched for a signal of function-specific introgression that might suggest concerted selection by using Gene Ontology (GO) analysis, the power of which is limited by the unknown but probably considerable proportion of hitchhiking genes. Separate GO analysis of the gene set acquired by each of the strains through introgression failed to yield overrepresented GO categories that were both reasonably specific and previously associated to wine fermentations ( Supplementary Data 3 ). However, when GO analysis was performed using the set of genes introgressed into any of the strains, the categories ‘GO:0006807: nitrogen compound metabolic process’ and ‘GO:0051171: regulation of nitrogen compound metabolic process’ were found to be overrepresented (corrected P values <0.05; Supplementary Data 3 ). Moreover, the use of a gene pool assembled so that the redundancy resulting from the presence of an introgressed gene in multiple strains was preserved, which highlighted the additional categories ‘GO:1900071: regulation of sulphite transport’, ‘GO:0006808: regulation of nitrogen utilization’, ‘GO:0019740: nitrogen utilization’, and ‘GO:0008238: exopeptidase activity’, among others ( Supplementary Data 3 ). These categories include genes pertinent to wine fermentation, some of which have been previously shown in S. cerevisiae wine strains to be involved in horizontal gene transfer (HGT) events [34] , [35] or genomic rearrangements [36] associated with anthropic environments. Some other overrepresented GO categories include one or several genes located close to genes relevant for nitrogen or sulphite metabolism and could possibly appear as overrepresented as a result of hitchhiking. All the introgressions on chromosome 2 harbour ASP1 , a gene encoding the cytosolic L-asparaginase used to degrade asparagine to be used as nitrogen source. This locus was previously associated with low acetic acid production in S. cerevisiae wine strains by quantitative trait loci (QTL) mapping [37] . Curiously, a similar gene induced by nitrogen starvation ( ASP3 ) was acquired by some S. cerevisiae strains by horizontal gene transfer [35] . Also, nine strains contained variably sized introgressions of subtelomeric regions of chromosome 7 that contained FZF1 ( Fig. 3 and Supplementary Data 2 ). This gene has been shown to encode a fast-evolving transcription factor that regulates several genes, including the gene encoding Ssu1, an efflux pump involved in sulphite resistance [38] . All introgressions in this set also encompass the ZRT1 gene that encodes a high-affinity zinc transporter that was recently reported to exhibit a sequence signature of balancing selection in S. cerevisiae [39] . Whereas the 900-bp sequence of the coding region of FZF1 is identical in all introgressed strains, it exhibits 16 and 126 SNPs when compared with reference strains of S. eubayanus and S. uvarum , respectively. Interestingly, the introgressed ZRT1 allele is highly diverged from both reference strains (149 and 148 SNPS, respectively). For both FZF1 and ZRT1 , there is no evidence of introgression from other known Saccharomyces species. In addition to differences in the coding region, the FZF1/ZRT1 intergenic region appears to carry a large insertion when compared with S. eubayanus ( Supplementary Fig. 4 ). Since only the S. cerevisiae copy of the FZF1 gene can be retrieved from the S. pastorianus genome, it is not possible to compare these introgressions to the S. eubayanus sub-genome of the hybrid species. We also searched for the presence of non- Saccharomyces fungal DNA using de novo assemblies constructed with the subset of reads that could not be mapped to the S. uvarum reference genome. Our searches did not reveal the presence of non- Saccharomyces open reading frames (ORFs), except for genes known to be present in three horizontally transferred regions previously identified in S. cerevisiae wine yeasts [34] and originating from yeasts outside this genus ( Supplementary Table 8 ). Since all the nine strains harbouring genes from these regions also had introgressions for other Saccharomyces species and all but one were associated with anthropic environments it is possible that non- Saccharomyces DNA was transmitted simultaneously with Saccharomyces introgressions. In Saccharomyces , several cases of genome modifications through hybridization [11] , introgression [31] , [32] , [40] , genome rearrangements [36] , [41] and HGT [34] , [35] have been documented, suggesting that genomes modified in this manner appear to be selected for in many industrial environments. Eloquent examples are the interspecies hybrids S. pastorianus ( S. cerevisiae × S. eubayanus ) in lager beer and S. cerevisiae × S. uvarum and S. cerevisiae × S. kudriavzevii in certain types of wines and of Belgian-style beers [13] , [14] , [15] . HGT events also appear to enhance the attributes of S. cerevisiae wine strains [34] , [35] . These changes have led to the domestication of Saccharomyces lineages as they have become genetically distinct from their wild relatives [6] , [42] , [43] in ways that are beneficial to humans. Although the process shares some similarities to what has been documented for plant crops and livestock [44] , HGT, interspecies hybridization and introgression provide a broader array of genetic mechanisms that lead to domesticated phenotypes. Here we present for the first time evidence of domestication in S. uvarum . In our study, we detected multiple introgressions, mainly of S. eubayanus genomic DNA, into the genomes of European wine or cider strains of S. uvarum . These introgressions were also found in S. uvarum × S. cerevisiae hybrids, which suggests that the S. eubayanus contribution is advantageous even in ‘enriched’ hybrid genomes. We postulate that the anthropic habitats colonized by S. uvarum in Europe may have favoured hybridization of S. uvarum with S. eubayanus , followed by subsequent introgression by backcrossing to S. uvarum . We suggest that hybrids or introgressed strains involving these two species may be less fit than the clean parental lineages in their natural South American habitat. Many S. cerevisiae wine strains possess three gene clusters acquired from non- Saccharomyces yeasts by HGT [34] . These regions are 120 kb long and include 34 genes, many of which are involved in key aspects of must fermentation such as the metabolism and transport of sugars and nitrogen. Hence, there seems to be some similarity between our findings in S. uvarum and those reported for S. cerevisiae because, in both cases, selective pressures in anthropic environments seem to have promoted genome adaptations involving interspecies exchange of genetic material. Nevertheless, the global pattern of domestication in S. cerevisiae seems to be different from that observed here in S. uvarum . The marked reduction of genetic diversity of S. cerevisiae wine domesticates relative to their wild relatives has no parallel in S. uvarum because the Holarctic wild and domesticated strains are indistinguishable in this respect. It is not clear if S. eubayanus introgressions occurred repeatedly or if they are the result of a single hybridization event that then spread throughout the European population. The latter possibility seems to be more in line with the apparent low abundance of S. eubayanus in Europe. The polymorphic pattern of the introgressions when different strains are compared suggests that their fixation or elimination from the population has not yet stabilized. Judging from the widespread occurrence of introgressed strains across Europe and their almost complete absence in wild populations, we hypothesize that introgressions are rapidly lost in European natural environments. This and other recent studies [12] , [45] concur in documenting an ancestral Nothofagus association for the two basal Saccharomyces species, S. eubayanus and S. uvarum . For S. eubayanus , two populations have also been reported in Patagonia, with a genetic divergence of 1% (ref. 46 ), that is similar to the divergence measured between the two Patagonian S. uvarum populations. In South America, S. eubayanus and S. uvarum share the Nothofagus niche, but S. eubayanus seems to be much more elusive than S. uvarum in the Northern Hemisphere. Only three isolates of S. eubayanus were recently reported in North America [46] , and the evidence presented here for the presence of S. eubayanus in Europe remains indirect. For S. uvarum , we could expand the association with Nothofagus by identifying a highly divergent population in New Zealand and Tasmania, which constitutes a significant addition to the diversity of early diverged Saccharomyces lineages found in the Southern Hemisphere. The partial reproductive isolation of the Australasian population is comparable to what is observed for the most divergent populations of S. paradoxus (32% spore viability) [30] and also fit within the range of results obtained for divergent lineages of S. cerevisiae found in China that have 10.2–55% spore viabilities [5] . Therefore, until more detailed analyses are carried out, we adopt a conservative view and regard the Australasian population as a considerably divergent S. uvarum population, possibly the result of an ongoing process of allopatric speciation. Although the two South American populations of S. uvarum are generally sympatric, their distribution ranges appear to only partially overlap. In fact, the distribution of one of these populations (SA-A) is restricted to the northern part of Patagonia, whereas the other population (SA-B) has a distribution that extends to southern Patagonia, including Tierra del Fuego ( Fig. 1c ). The evidence for admixture that we obtained and the minor contributions from population SA-B in all studied isolates from population SA-A revealed in the STRUCTURE analysis ( Fig. 1d ) suggest that the two populations are presently in contact and that there is little or no relevant reproductive isolation between them, which could be experimentally confirmed. The geographic distribution of the two Patagonian populations can be related to the phylogeography of Nothofagus whose species tend to have latitudinally disjunct populations as a consequence of long-lasting vicariance events related to past glaciations and to the presence of an ancient paleobasin at mid-latitudes in Patagonia [45] , [47] , [48] . Our results fit this model of two, historically isolated clades, one in the north and the other in the south. Favourable climatic and geologic conditions prevailing since 25,000 years ago seem to have facilitated secondary contact. In mid-latitudes, northward migration of Nothofagus appears to have been more efficient than southward migration [48] , which is concordant with what we have observed for S. uvarum ( Fig. 1c ). Phylogenomic and population structure analyses support the view that a restricted subset of population SA-A gave rise to the Holarctic population, although vectors and mechanisms of this migration into the Northern Hemisphere remain to be elucidated. The lack of diversity found in the extant residents of the Northern Hemisphere contrasts with the vast geographical area colonized, which ranges from temperate North America to Europe and Asia, and suggests that the subsequent dispersal across these northern continents occurred rapidly enough to prevent the accumulation of many local mutations. Australasia and South America harbour the only ecosystems where Nothofagus trees can be found presently and were once united in the mega-continent Gondwana. We propose that the much higher genetic diversity of both S. uvarum and S. eubayanus found in the Southern Hemisphere, the high frequency of isolation and the Nothofagus association suggest that both species are native to the Southern Hemisphere and that their primal niche is the Nothofagus system. Based on the basal position of the S. uvarum/S. eubayanus lineage, it seems plausible to hypothesize that the last common Saccharomyces ancestor thrived in the Southern Hemisphere in association with the Nothofagus system. In this scenario, an early derived lineage may have undergone speciation while associated with Nothofagus , originating S. eubayanus and S. uvarum , whereas another lineage may have migrated to the Northern Hemisphere through Southeast Asia, the only region of the globe where southern beech and oak relatives of the Fagaceae overlap [49] . The transition to the oak system could have been associated with the formation of other species, giving rise to endemic Asian taxa such as S. arboricola and S. mikatae , as well as to species with more global Holarctic distributions, such as S. kudriavzevii, S. paradoxus and S. cerevisiae . Yeast isolation, identification and crosses The selective protocol used for Saccharomyces isolations was based on the selective enrichment in a raffinose–ethanol liquid medium as previously described [4] , [12] . Putative Saccharomyces isolates were confirmed by the observation of Saccharomyces -type ascospore production. Species identifications were based on DNA sequencing of the ITS and D1/D2 regions of the rDNA. For each pair of strains tested, ascospores were isolated and crossed to obtain intra- and interspecies hybrids. Hybridization between the two parental strains was confirmed by sequencing of the MET2 and/or FSY1 genes and confirmation of the expected heterozygous sites. For each cross, interspecific spore viability was determined by examining at least 200 ascospores produced by two independent hybrid strains. Quality filtering and alignment to reference genomes Genomic Illumina sequencing libraries were prepared for most of the isolates (or their monosporic derivatives; Supplementary Table 1 ) and sequenced for 100 cycles (single-end) or 2 × 100 cycles (paired-end) using the Illumina HiSeq2000 or GAxII systems. Some strains were multiplexed as described previously [33] . To make results directly comparable, all sequencing data were treated as single-end reads. Reads were filtered to include only those with a perfect index match. To optimize downstream analysis, quality control for each set of reads was carried out using FASTX toolkit v0.13.2 ( http://hannonlab.cshl.edu/fastx_toolkit/ ). In brief, any adapter sequences were clipped from the reads, and low quality bases from the 3′-end of reads were trimmed based on the Illumina Phred scores. Reads were retained only if read length was above 32. Finally, reads were discarded if >5% of the positions had Phred scores <10. Filtered reads from each isolate were mapped to the reference genome of S. uvarum CBS 7001 (ref. 50 ) using SMALT v0.6.4 (Wellcome Trust Sanger Institute, www.sanger.ac.uk/resources/software/smalt/ ) with default parameters, except that we allowed for a step size of 2 (−k 13–s 2) and SAM format output. In addition to reporting the best gapped alignment for each read, the default settings of SMALT v0.6.4 only generate uniquely mapped reads. Downstream analyses, such as conversion to BAM format, sorting, indexing, several mapping statistics and consensus genotype calling were performed using the tools available in the SAMtools package v1.18 (ref. 51 ) with the default parameters. Consensus genotypes in VCF format were then converted to fastq format by restricting the maximum depth to 100, 250 or 500, depending on the median mapping depth, in order to avoid overrepresented regions that could be copy-number variants or artefacts. A fasta file was generated for each alignment where base calls with a consensus Phred quality score <40 (equivalent to a 99.99% of base call accuracy) were masked to lower case. The final quality of the filtered consensus fasta files was assessed by calculating the proportion of high-quality bases (with Phred quality score >40, Q40 hereafter) relative to the entire mapped genome. For downstream analysis, all bases with Phred quality score <Q40 were converted to an ‘N’. The resulting fasta files were pooled together to generate multiple sequence alignments for each reference contig. Reads from the three hybrid strains studied and from S. bayanus NCAIM 676 ( Supplementary Table 1 ) were treated in the same way as described above but were mapped to a combined reference that included the genomes of S. uvarum CBS 7001, S. kudriavzevii IFO 1802 (ref. 50 ) and S. cerevisiae (UCSC version sacCer3). This process provided a reliable alignment of the mappable portion of reads for each hybrid strain to the S. uvarum reference genome that were treated in the same way as for the other isolates. Phylogeny, population structure and polymorphism analyses Before analyses, regions with evidence for introgression of S. eubayanus (see below) were removed from the alignments. For phylogenetic and population structure analyses, unambiguous SNPs were extracted from the contig multiple sequence alignments if the evaluated site was represented only by high-confidence alleles, meaning that for each position information was available for all of the isolates. Two phylogenetic analyses were carried out for our strain data set. The first included the complete set of isolates and was constructed based on the concatenated SNP alignment of chromosomes 5, 8 and 12 (3,113 SNPs; note that chromosome 10 was mislabeled as chromosome 12, and vice-versa, in the annotation of Scannell et al [50] ). A more restricted phylogeny was built using the 54 isolates that exhibited >70% of Q40 bases. Chromosomal SNPs were then concatenated to generate a whole-genome SNP alignment (129,096 SNPs). Both phylogenies were inferred by the Neighbour-Joining method with 1,000 bootstrap replicates using the p -distance to compute evolutionary distances. S. eubayanus CRUB 1568 was used as outgroup. Phylogenetic analyses were performed in MEGA5 (ref. 52 ). For the restricted data set, a maximum likelihood phylogeny was also performed using the rapid bootstrap algorithm in RAxML [53] with GTRCAT approximation. Population structure of S. uvarum was explored using the model-based Bayesian clustering method implemented in STRUCTURE v2.3.4 (ref. 54 ). For the global sampling of S. uvarum , STRUCTURE was run with a subset of 10,337 equally spaced SNPs. The divergent Australasian population was then removed to facilitate identification of subtle population structure among the remaining clades of S. uvarum . A new subset of 9,391 equally spaced SNPs was generated for this data set. For both data, the value of K was allowed to vary from K =1 to 8, and the number of Markov chain Monte Carlo iterations was set to an initial burn-in period of 50,000 iterations, followed by 30,000 iterations of sampling. Allele frequencies were assumed to be correlated among populations, and the ancestry model allowed for admixture. Ten independent simulations were run for each value of K and stability was assessed by monitoring the s.d. between simulations. The optimal number of K clusters were estimated from the ad hoc statistic Δ K [55] . CLUMPP v1.1.2 (ref. 56 ) was used to compute the similarity coefficient between replicate simulations of STRUCTURE ( G ′) using the Greedy or LargeKGreedy ( K =7 and 8) algorithms with 10,000 random configurations. The highest value of H ′ was always found to be above 0.99, indicating high modal similarity between the replicate Q-matrices. Nucleotide diversity within populations and divergence between populations were estimated using Variscan v2.0 (ref. 57 ). Only positions with valid alleles in at least 90% of the individuals were used for calculations (defined with the NumNuc parameter together with CompleteDeletion=0 and FixNum=1). The null distributions of Tajima’s D statistic were generated in ms [58] under the standard coalescent neutral model with 10,000 independent simulations conditioned on the sample size (as determined by NumNuc in Variscan) and observed estimates of θ W . Sliding window analyses were performed on non-overlapping windows of 1,000 sites, retaining only those windows where at least 500 sites (Q40) were used in calculations. Statistics of shared polymorphisms, fixed differences and private alleles were calculated using sharedPoly programme from the analysis package ( http://molpopgen.org/ ) [59] using whole-genome SNP alignments. Bayesian coalescent analysis Rooted coalescent phylogenies were estimated using a subset of strains from each identified population. Potential hybrid/mosaic strains were excluded from the original alignments in order to minimize violations of the models’ assumptions. High-confidence alignment sites were extracted from the contig alignments whenever a site was represented with an unambiguous high-quality allele (Q40) in all strains. These high-confidence alignments were broken into regions with no four-gamete-test violations using RminCutter.pl v1.05 ( https://github.com/RILAB/rmin_cut/ ) [60] with the following settings: -v -q -f -m -g -n. For each contig, the segment with the highest number of polymorphisms was chosen and used as a different partition in the BEAST v1.7.4 package [61] . This approach produced a total of 51,159 sites with 2,884 segregating positions. BEAST was run with linked partitions using the coalescent constant size tree prior, the GTR+Γ+I model of sequence evolution and a strict molecular clock. Monophyly was assumed for the main clades. Coalescent estimates are given in units of substitution per site. Two independent chains of 30,000 Markov chain Monte Carlo generations each were performed, with sampling at every 1,000 generations. Traces were combined in LogCombiner, discarding the first 10% of generations as burn-in, and convergence was assessed by examination of the effective sampling size in Tracer v1.5.0. All estimated parameters showed effective sampling size values >600. Phylogeny of the genus Saccharomyces We deployed a recent multi-locus sequence approach [62] to examine the evolutionary relationships among the species and known populations of the genus Saccharomyces , including the new Australasian population of S. uvarum described here. Complete coding sequences for the 14 genes were extracted from the available annotations of six Saccharomyces species [50] , [63] , ( Saccharomyces Genome Database). Homologous regions for a representative strain of the Far Eastern (IFO 1804) and North American (YPS 138) populations of S. paradoxus were retrieved from the BLAST server available at http://www.sanger.ac.uk/cgi-bin/blast/submitblast/s_paradoxus_sgrp/ [6] . A local BLAST database was also set to retrieve the same regions from our de novo assemblies (see below) of S. eubayanus (CRUB 1568) and from one representative strain of the S. uvarum Australasian population (ZP 962), and from the reference genome of Naumovozyma castellii CBS 4309 (NCBI assembly ASM23734v1), which was used as an outgroup. The 14 coding sequences were concatenated and then aligned with FSA v1.15.7 (ref. 64 ). Sites with alignment gaps and unknown bases were removed from the alignment before phylogenetic reconstruction. A maximum likelihood phylogeny was estimated in PhyML v3.0 (ref. 65 ) using the GTR+Γ+I model of sequence evolution, estimating the Γ distribution parameter, with five substitution rate categories, and the proportion of invariable sites. Tree topology moves were performed using the best of NNI and SPR searches with five initial random trees. Branch support was estimated with 100 non-parametric bootstrap replicates. Screening for foreign genes in the genomes of S. uvarum We searched for evidence of introgressions from other Saccharomyces species by mapping the reads to a combined reference including all the available annotated coding sequences of six Saccharomyces species [50] , [63] , ( Saccharomyces Genome Database). Reads were quality-filtered as above and mapped to this combined reference using BWA with default parameters [66] . SAMtools v1.18 (ref. 51 ) was used for the manipulation of the resulting BAM files, following the same approach as described above. Genes showing >80% of Q40 bases, which provides a good initial measure for the mappability of reads to the corresponding targets, in >100 bases were selected for further analysis. Finally, only genes with orthologues unambiguously annotated in at least four species, including S. uvarum , were analysed. Exceptions are mainly owing to the fact that some of the bona fide transfers of genes that are not annotated in S. uvarum genome seemed to be close neighbours to other genes that are annotated in both the S. uvarum and donor genomes ( Supplementary Data 1 ). A gene was recognized as having a foreign origin if the number of reads that mapped to the putatively donor genome was higher than the sum of the reads that mapped to the orthologous genes in the other Saccharomyces species. Five single-gene transfer events were identified using this process but were excluded from further analysis because they corresponded to short coding sequences (<200 bp long) or had a low number of reads mapped. Introgressions from other fungal non- Saccharomyces species were searched by assembling the reads that failed to map to the reference genome of S. uvarum into contigs with Velvet v.1.2.08 (ref. 67 ). Assembled contigs with >500 bp length were used as query and ‘blasted’ against the ORF sequences of the three horizontally transferred regions identified by Novo et al . [34] and to the NCBI nr database using BLASTN (1e–10e value cutoff). Only the best blast hit for each query was retained and hits to the rDNA region were excluded from the analysis. Screening for introgressions from S. eubayanus S. eubayanus does not yet have a reference assembly against which reads can be mapped. We generated additional reads from the type strain of S. eubayanus (CRUB 1568) in this study, and the corresponding reads were treated with the methods described above for the alignment to the reference genome of S. uvarum . Pairwise divergence between the S. uvarum and S. eubayanus type strains was used as a proxy to search for evidence of DNA segments of S. eubayanus in the genomes of S. uvarum . Divergence per site, k , (with Jukes–Cantor correction) was calculated in Variscan v2.0 (ref. 57 ) using a non-overlapping sliding window of 1,000 sites. Only the windows with at least 500 high-quality sites used in the pairwise comparisons (Q40) were retained for further analyses. For easier visualization and interpretation of these results, each data point in the plots ( Fig. 2 ) represents the average divergence of itself plus three windows on each side. GO analysis Standard GO term discovery was performed with the Generic GO Term Finder [68] , [69] . This procedure, however, does not consider the observation that the same gene can be found within introgressed regions of multiple strains. To account for this redundancy, we first determined the number of times each GO attribute was annotated for the set of introgressed genes in each strain and then summed over all the strains considered. Fisher’s exact test was used to test the hypothesis that a specific GO attribute was overrepresented in the pooled introgressed gene set relative to the expected number of genes in the reference gene annotation file (retrieved from YeastMine on December 2013). The Bonferroni procedure was applied to correct for multiple comparisons using the total number of tests performed for each ontology term (process, component or function). Significance was assessed for all data with a corrected P value cutoff of 0.05. De novo assemblies and analysis of FZF1 and ZRT1 sequences For a more detailed analysis of the introgression on chromosome 7, which harbours FZF1 and ZRT1 , we performed de novo genome assemblies of the Illumina single-end or paired-end reads for all strains included in this study, using Velvet v.1.2.08 (ref. 67 ). The expected coverage for each region was calculated, and the contigs with a coverage value <10 × were discarded, whereas the regions with a coverage value <15 × were masked. To retrieve the gene sequences, we set up a local BLAST database for each genome and searched for the aforementioned genes by a TBLASTX search using the S. uvarum FZF1 and ZRT1 sequences from strain CBS 7001 ( Saccharomyces Genome Database) as queries (PORF 7762; PORF 7764). The gene sequences were then aligned using MEGA v.5.05 (ClustalW) [52] . For the promoter analysis of each gene, a 1,000-bp upstream sequence was retrieved from SGD and the aforementioned procedure was followed. How to cite this article : Almeida, P. et al . A Gondwanan imprint on global diversity and domestication of wine and cider yeast Saccharomyces uvarum . Nat. Commun. 5:4044 doi: 10.1038/ncomms5044 (2014). Accession codes: The sequencing data generated in this study have been deposited in the National Center for Biotechnology Information short-read archive (NCBI-SRA) under accession codes PRJNA230139 and PRJEB5133 .